Multisensory training reverses midbrain lesion-induced changes and ameliorates haemianopia Failure to attend to visual cues is a common consequence of visual cortex injury. Here, we report on a behavioural strategy whereby cross-modal (auditory–visual) training reinstates visuomotor competencies in animals rendered haemianopic by complete unilateral visual cortex ablation. The re-emergence of visual behaviours is correlated with the reinstatement of visual responsiveness in deep layer neurons of the ipsilesional superior colliculus (SC). This functional recovery is produced by training-induced alterations in descending influences from association cortex that allowed these midbrain neurons to once again transform visual cues into appropriate orientation behaviours. The findings underscore the inherent plasticity and functional breadth of phylogenetically older visuomotor circuits that can express visual capabilities thought to have been subsumed by more recently evolved brain regions. These observations suggest the need for reevaluating current concepts of functional segregation in the visual system and have important implications for strategies aimed at ameliorating trauma-induced visual deficits in humans. Countless times each day, we orient our eyes to objects of interest and importance. This seemingly effortless ability depends on interactions between the phylogenetically older midbrain superior colliculus (SC) and the more recently evolved visual cortex. Disrupting descending corticotectal inputs attenuates the visual responsiveness of deep SC neurons [1] and produces an enduring contralesional haemianopia [2] , [3] . However, the physiological changes in the SC and the lack of SC-mediated behavioural responses to contralesional visual stimuli following cortical disruption are surprising in light of the remaining visual inputs to the SC from retina and other visually responsive structures [4] , [5] . Yet many visual neurons in the deep SC also are multisensory and normally respond to both auditory and visual stimuli [6] . These SC neurons integrate cross-modal cues so that a concordant auditory stimulus enhances their visual responsiveness [7] , [8] , [9] , [10] , [11] and facilitates the orientation behaviours they subserve [12] , [13] , [14] . Recently, the visual responses of deep SC neurons have been shown to be plastic in intact adult animals, with some visually unresponsive neurons becoming responsive to visual stimuli following repeated exposure to cross-modal cues [15] , [16] . Therefore, we posited that purposeful behavioural interactions with cross-modal cues might enhance the effectiveness of visual SC inputs in cortically lesioned animals, thereby rendering midbrain neurons visually responsive and once again capable of supporting visual orientation behaviours. We tested this possibility by training haemianopic cats in a task requiring repeated, food-rewarded orienting movements to a salient auditory cue presented together with a spatially and temporally coincident (but task irrelevant) visual cue delivered at a single peripheral location within the anopic hemifield. We then assayed the behavioural consequences of this strategy and determined its neural correlates in the SC, before, and following, this rehabilitative training. Here we report that such training reinstates basic visuomotor competencies within several weeks by facilitating the re-emergence of visual activity in the deep (for example, multisensory layers) of the SC via training-induced alterations to inputs that these neurons receive from lesion-spared regions of association cortex. Mongrel cats ( n =20) were trained in a standard visual orientation task ( Fig. 1a ) to orient to, and approach, a visual cue presented between 105° left and right of central fixation (0°) (ref. 17 ). Following surgical recovery from unilateral extirpation of all contiguous areas of visual cortex ( Supplementary Fig. 1 ), post-lesion testing revealed a profound and persistent contralesional haemianopia ( Figs 2a and 3a,b ). In most cases, transient contralesional auditory and tactile deficits were noted post-operatively, but these resolved within 2–10 days, with animals displaying no obvious auditory or somatosensory deficits thereafter. Contralesional visual orientation deficits persisted for periods up to 21 months (range=3–21 months). During this period, and before initiating cross-modal training, orientation in the haemianopic field was completely absent in all lesioned animals. Despite the extensive exposure to contralesional visual cues during post-lesion testing sessions, the animals showed an apparent lack of awareness of these stimuli and failed to react in any discernible way to their presentation. 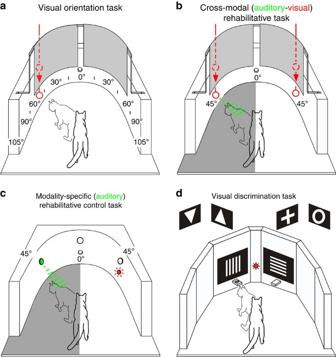Figure 1: Four experimental behavioural tasks used. (a) Animals were trained to fixate (0°) and then orient to visual cues introduced suddenly into the visual field quasi-randomly at each 15° of visual eccentricity. Food rewards for correct orientation were delivered at that eccentricity. During catch trials (no cue delivered) and for trials in which the cue was not responded to, animals moved straight ahead to receive food rewards at fixation. On reaching the criterion (95% averaged across eccentricities), all contiguous visual cortex was removed unilaterally, and animals were retested to verify an enduring contralesional haemianopia. (b) For cross-modal training, animals made repeated food-rewarded orienting movements to a spatiotemporal coincident auditory–visual cue presented at 45° in the anopic hemifield (grey area). The same arena was used for both orientation testing and cross-modal training. Cross-modal cues were generated by sliding a white ball along the wall of the chamber. To preclude anticipatory movements, on some trials a visual cue was presented alone at 45° in the intact hemifield. Food rewards were delivered at site of cue presentation. If no cue was delivered, animals moved towards fixation point for food rewards. (c) As a control for the cross-modal task, animals made orientations to auditory cues presented alone at 45° into the anopic hemifield (grey shaded area). Computer-generated cues were delivered by a speaker and approximated the intensity and duration of auditory cues used for cross-modal training. To minimize visual cues during testing, training was conducted in a darkened room. Speakers were covered with black speaker grill cloth to provide a uniform background that further minimized visual cues. On select trials, visual cues were presented alone at 45° in the intact hemifield. (d) To evaluate visual capabilities beyond orientation, some animals also were trained pre-operatively in a forced-choice paradigm to discriminate vertical versus horizontal gratings of different spatial frequencies and simple form discrimination (triangle orientation; cross versus annulus). Computer-generated white-on-black background discriminanda were presented on two flat screen LCDs positioned 15° eccentric to central fixation. The animal fixated on a central fixation point and was rewarded for correct movements toward the selected ‘correct’ discriminanda where food rewards were delivered. Figure 1: Four experimental behavioural tasks used. ( a ) Animals were trained to fixate (0°) and then orient to visual cues introduced suddenly into the visual field quasi-randomly at each 15° of visual eccentricity. Food rewards for correct orientation were delivered at that eccentricity. During catch trials (no cue delivered) and for trials in which the cue was not responded to, animals moved straight ahead to receive food rewards at fixation. On reaching the criterion (95% averaged across eccentricities), all contiguous visual cortex was removed unilaterally, and animals were retested to verify an enduring contralesional haemianopia. ( b ) For cross-modal training, animals made repeated food-rewarded orienting movements to a spatiotemporal coincident auditory–visual cue presented at 45° in the anopic hemifield (grey area). The same arena was used for both orientation testing and cross-modal training. Cross-modal cues were generated by sliding a white ball along the wall of the chamber. To preclude anticipatory movements, on some trials a visual cue was presented alone at 45° in the intact hemifield. Food rewards were delivered at site of cue presentation. If no cue was delivered, animals moved towards fixation point for food rewards. ( c ) As a control for the cross-modal task, animals made orientations to auditory cues presented alone at 45° into the anopic hemifield (grey shaded area). Computer-generated cues were delivered by a speaker and approximated the intensity and duration of auditory cues used for cross-modal training. To minimize visual cues during testing, training was conducted in a darkened room. Speakers were covered with black speaker grill cloth to provide a uniform background that further minimized visual cues. On select trials, visual cues were presented alone at 45° in the intact hemifield. ( d ) To evaluate visual capabilities beyond orientation, some animals also were trained pre-operatively in a forced-choice paradigm to discriminate vertical versus horizontal gratings of different spatial frequencies and simple form discrimination (triangle orientation; cross versus annulus). Computer-generated white-on-black background discriminanda were presented on two flat screen LCDs positioned 15° eccentric to central fixation. The animal fixated on a central fixation point and was rewarded for correct movements toward the selected ‘correct’ discriminanda where food rewards were delivered. 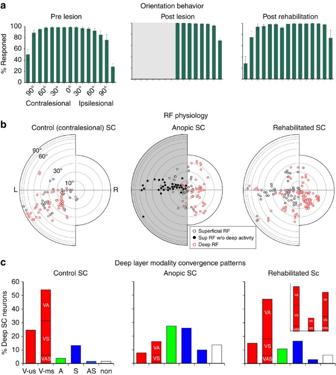Figure 2: Behavioural performance and physiological correlates after cross-modal rehabilitation of lesion-induced visual deficits. (a) Cumulative histograms show the mean visual orientation performance (±s.e.m.) of animals tested with stimuli at each 15° of eccentricity along the azimuth in both hemifields before unilateral visual cortex ablation (left), following the lesion (center) and after cross-modal rehabilitative training (right). Similar pre-lesion and post-lesion profiles were apparent in all animals but data shown here are only for those (n=11) that underwent rehabilitative training. Note the complete absence of responses to visual cues throughout the contralesional hemifield (center). Although either the right or left visual cortex was ablated, here the anopic hemifield is normalized to left visual space. (b) The position of visual RFs centres of superficial (black circles) and deep (red circles) layer SC neurons recorded in three different experimental conditions is plotted on polar coordinate representations of left (L) and right (R) visual space. Concentric circles represent radial coordinates from central visual space, and vertical and horizontal lines represent the respective meridians. All data were normalized to the left hemifield to facilitate comparisons. Left figurine: the distribution of visual RFs recorded in the control (that is, contralesional) SC of two animals. Middle figurine: recordings in the ipsilesional SC of four haemianopic animals revealed that while superficial layer visual responses could be evoked and contralesional activity was present in these animals following visual cortex removal, deep layer visual responsiveness was severely compromised. Moreover, there were numerous electrode penetrations through the superficial layers that did not have corresponding visual activity in their underlying deep layer neurons (filled black circles). There also was now an anomalous visual representation in central visual space that extended into the opposite hemifield. Right: cross-modal training reinstated deep layer visual responsiveness in the contralesional hemifield but the anomalous central representation was retained. (c) Deep layer modality convergence patterns in: control SC (left); ipsilesional SC before (middle) and after (right) cross-modal training. Note that the training-induced re-emergence of visual responsiveness was greatest among multisensory neurons. A, auditory; non, non-responsive; S, somatosensory; V, visual; V-u, visual (unisensory); V-m, visual (multisensory). Full size image Figure 2: Behavioural performance and physiological correlates after cross-modal rehabilitation of lesion-induced visual deficits. ( a ) Cumulative histograms show the mean visual orientation performance (±s.e.m.) of animals tested with stimuli at each 15° of eccentricity along the azimuth in both hemifields before unilateral visual cortex ablation (left), following the lesion (center) and after cross-modal rehabilitative training (right). Similar pre-lesion and post-lesion profiles were apparent in all animals but data shown here are only for those ( n =11) that underwent rehabilitative training. Note the complete absence of responses to visual cues throughout the contralesional hemifield (center). Although either the right or left visual cortex was ablated, here the anopic hemifield is normalized to left visual space. ( b ) The position of visual RFs centres of superficial (black circles) and deep (red circles) layer SC neurons recorded in three different experimental conditions is plotted on polar coordinate representations of left (L) and right (R) visual space. Concentric circles represent radial coordinates from central visual space, and vertical and horizontal lines represent the respective meridians. All data were normalized to the left hemifield to facilitate comparisons. Left figurine: the distribution of visual RFs recorded in the control (that is, contralesional) SC of two animals. Middle figurine: recordings in the ipsilesional SC of four haemianopic animals revealed that while superficial layer visual responses could be evoked and contralesional activity was present in these animals following visual cortex removal, deep layer visual responsiveness was severely compromised. Moreover, there were numerous electrode penetrations through the superficial layers that did not have corresponding visual activity in their underlying deep layer neurons (filled black circles). There also was now an anomalous visual representation in central visual space that extended into the opposite hemifield. Right: cross-modal training reinstated deep layer visual responsiveness in the contralesional hemifield but the anomalous central representation was retained. ( c ) Deep layer modality convergence patterns in: control SC (left); ipsilesional SC before (middle) and after (right) cross-modal training. Note that the training-induced re-emergence of visual responsiveness was greatest among multisensory neurons. A, auditory; non, non-responsive; S, somatosensory; V, visual; V-u, visual (unisensory); V-m, visual (multisensory). 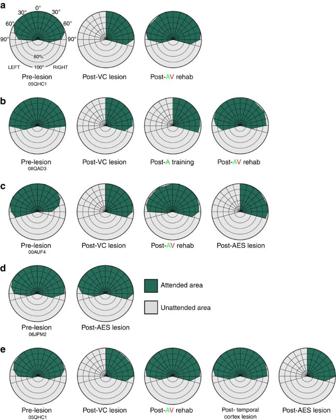Figure 3: Polar plots of the visual orientation capabilities of five representative animals following visual cortex lesions, cross-modal training and other experimental manipulations. (a) Post-lesion training with cross-modal auditory–visual (AV) cues ameliorated visual cortex lesion-induced haemianopia. (b) By contrast, post-lesion training with auditory cues (A) alone failed to mediate recovery. Subsequent training with cross-modal cues, however, reinstated visual orientation in the previously anopic hemifield. (c) Visual orientation competencies reinstated by cross-modal training were lost following lesions of AES cortex. (d) Despite the importance of AES for visual orientation in rehabilitated animals, AES lesions had no effect on visual orientation capabilities in normal animals. (e) Reinstated visual orientation competencies were not affected by non-AES cortical lesions. Full size image Figure 3: Polar plots of the visual orientation capabilities of five representative animals following visual cortex lesions, cross-modal training and other experimental manipulations. ( a ) Post-lesion training with cross-modal auditory–visual (AV) cues ameliorated visual cortex lesion-induced haemianopia. ( b ) By contrast, post-lesion training with auditory cues (A) alone failed to mediate recovery. Subsequent training with cross-modal cues, however, reinstated visual orientation in the previously anopic hemifield. ( c ) Visual orientation competencies reinstated by cross-modal training were lost following lesions of AES cortex. ( d ) Despite the importance of AES for visual orientation in rehabilitated animals, AES lesions had no effect on visual orientation capabilities in normal animals. ( e ) Reinstated visual orientation competencies were not affected by non-AES cortical lesions. Full size image To determine the neurophysiological correlates of the haemianopia, single-neuron recording experiments were conducted in animals ( n =4) with persistent deficits (see Methods). Electrode penetrations into the control (contralesional) SC ( Supplementary Fig. 2 ) revealed the typical distribution of visually responsive neurons in both its superficial (visual) and deep (multisensory) layers [4] , [6] . The latter receive converging input from cortex [18] and are directly involved in visual orientation via descending projections to brainstem motor areas [19] , [20] . Visual, auditory, somatosensory and multisensory neurons were evident [21] with visual receptive field (RF) centres restricted to contralateral visual space and organized into a topographical map that was in good register with the non-visual maps in these layers and with the overlying superficial layer visual map [6] . By contrast, recordings in the ipsilesional SC revealed a dramatic loss of visual activity when the electrode was advanced into the multisensory layers. Here neurons were no longer responsive to visual stimuli in large portions of the anopic field as shown in the individual example provided in Supplementary Fig. 2a and the population results shown in Fig. 2b (middle). The visually responsive neurons that were encountered in the multisensory layers were restricted to the most rostral aspects of the structure. Most of these neurons had their RF centre across the vertical meridian and were thus located in the ‘wrong’ (that is, ipsilesional) hemifield. Their RFs were displaced nasal to their overlying superficial layer counterparts (mean=13.47°; s.d.=±11.71°). In general, the lesion appeared to result in the selective elimination of visual responsiveness from much of the deep SC, thereby silencing unisensory visual neurons in those regions and rendering their multisensory counterparts insensitive to visual inputs ( Fig. 2c middle). In short, neurons in these layers were no longer able to support visual orientation behaviours (see, for example, Fig. 2a middle and Fig. 2b middle), yet appeared fully capable of robust responses to non-visual (that is, auditory and/or tactile) cues, reflecting a selective physiological loss consistent with the selective loss of visually guided behaviour. To determine if the lesion-induced visual orientation deficits could be ameliorated by cross-modal (auditory–visual) training, haemianopic animals ( n =11) were required to orient to and approach a spatiotemporally coincident auditory–visual cue presented at a single site on the azimuth, 45° into the haemianopic field ( Fig. 1b ). Daily rehabilitative training (5 × per week) consisted of 45–60 cross-model cue presentations interleaved with 10 visual cue presentations at the homologous location in the opposite (normal) hemifield, and 10 ‘catch trials’ in which no cue was delivered. After 4 weeks of training, all animals had regained orientation capabilities to visual cues presented at any eccentricity in the previously neglected hemifield. All rehabilitated animals retained this recovered capability without further cross-modal training until the end of the testing period (range=12–21 months). Post-mortem histological examination revealed that cortical ablation produced profound retrograde degeneration of the ipsilesional lateral geniculate nucleus ( Fig. 2b ). Taken together, these data suggest that the cross-modal training reinstated visuomotor competency by pathways independent of the lateral geniculate nucleus. To detail the spatiotemporal dynamics of the recovery process, haemianopic animals ( n =4) were evaluated before, immediately following, and 1 h after each rehabilitative session. Typically, visual orientation behaviour to stimuli in the compromised hemifield became evident after 9–11 days of cross-modal training ( Supplementary Fig. 3 ). Surprisingly, however, in every instance, the initial re-emerging orientations occurred to cues delivered within 30° of fixation rather than at the locus of the cross-modal training cue (that is, 45°). The recovery process was dynamic after a given session both in terms of the effective locations and the reliability of the responses to those locations. In the early stages of recovery, orientation responses were highly labile such that cues presented at a given location would be effective immediately after a cross-modal training session but then become ineffective 1 h later. However, with continued training, orientation capabilities were retained for longer periods following a session, and finally extended to successive daily sessions. The reinstatement of visual orientation also was progressive, beginning, as noted above, at a location nasal to the location of the training cue and then expanding in a central-to-peripheral manner until cues delivered at all eccentricities in the previously anopic hemifield were effective. These data indicate that labile, short-term alterations in the efficiency of visuomotor transformations during recovery are progressively instantiated with continued cross-modal training. To examine the possibility that an auditory cue presented alone would have the same rehabilitative effect, haemianopic animals ( n =2) were trained in the same paradigm, but now only the auditory cue was presented at the training location ( Fig. 1c , see also Methods). After 4 weeks ( n =1) or 6 weeks ( n =1) of this unisensory training, in which more than twice the number of auditory trials than required for recovery with cross-modal training were presented, neither animal showed evidence of recovery. The data from one of these animals is provided in Fig. 3b , which also show that subsequent cross-modal training with the typical number of training sessions/trials did induce recovery in this animal. The same was true of the second animal. These observations revealed that the coupling of the auditory and visual stimuli into a cross-modal configuration produced rehabilitative changes that were not replicated by using an auditory cue to initiate overt responses in the anopic hemifield. To explore the neurophysiological correlates of the recovery, recordings were made in the ipsilesional SC of rehabilitated animals ( n =4). Unlike the dramatic loss of visual activity in the multisensory layers that was typical of most electrode penetrations before cross-modal training, all ( n =50/50) penetrations made in these animals following cross-modal training yielded responses similar to those in normal animals. Neurons were encountered that responded to stimuli at various eccentricities (0–105°) throughout the previously anopic hemifield ( Fig. 2 ; see also Supplementary Fig. 2b ), but also evident was the retention of the anomalous representation in the ipsilesional hemifield discussed above. RF sizes had not changed from that in the control group (2,134±1,197°2 versus 2,545±1,664°2, respectively, P =0.18, F(1,147)=1.78, analysis of covariance controlling for horizontal and vertical eccentricity). Furthermore, the incidence of visually responsive neurons was similar to that in the opposite (control) SC, but the re-emergence of visual responsiveness was disproportionately higher among multisensory neurons ( Fig. 2c ). This suggests that the rehabilitative effects were exerted primarily on the multisensory architecture of the SC, presumably through multisensory integration, which can enhance the responsiveness of these neurons to visual cues [15] , [16] . Multisensory neurons displaying enhancement and depression were evident in these animals ( Supplementary Fig. 4 ). SC multisensory integration [18] , [22] and multisensory orientation behaviours [13] are known to depend on influences from association cortex, particularly the anterior ectosylvian sulcus (AES) [22] . Sensory neurons in this region are highly sensitive to experience [23] , [24] , [25] and may have been altered to assume a role in visual orientation in which they normally are not involved. To test this possibility, the effect of removing AES on SC-mediated visuomotor behaviour was examined in rehabilitated animals ( n =2) ∼ 3 months following cross-modal training. An example of the AES lesion is provided in Supplementary Fig. 1a . In both cases, visual orientation competencies were eliminated, reestablishing the contralesional haemianopia ( Fig. 3c ). By contrast, comparable lesions of AES in normal animals ( n =3) had no such effect on visual orientation ( Fig. 3d ). In a third rehabilitated animal, ablation of other regions in that hemisphere (that is, temporal cortex) failed to reinstate the haemianopia, but the haemianopia was re-established in that animal by subsequent removal of AES ( Fig. 3e ). Taken together, these data support the notion that cross-modal training induced changes in the multisensory circuitry of the SC via its inputs from AES, enabling SC-mediated visuomotor behaviours in the absence of visual cortex. To provide a physiological test of this hypothesis, recordings were made from visually responsive neurons ( n =59) in the ipsilesional SC of rehabilitated animals ( n =2) during cryogenic deactivation of AES (see Methods). As predicted, the overall deep layer visual activity was markedly degraded. However, K-means analysis of pre- versus post-deactivation visual responsiveness in these neurons revealed distinct neuronal populations as a function of their RF eccentricity ( Fig. 4d ). Neurons in the rostral SC, whose RFs represented the most central region of visual space, were least dependent on AES input and their visual responses were either moderately attenuated (mean reduction=18%) or enhanced (mean enhancement=30%) by AES deactivation. This was consistent with the observation that visual cortex-lesioned animals responded to visual stimuli at 0° even without rehabilitation. By contrast, all (26/26) of the neurons in caudal SC with RFs centres >15° (representing anopic regions of visual space before rehabilitation) were strongly depressed (mean reduction=84%) by AES deactivation. The vast majority (92.3%, 24/26) of these neurons were multisensory. The incidence and levels of visual response depression noted in these neurons was far greater than that reported in intact cats [22] , [26] , indicating that their dependence on inputs from AES had become markedly greater after cross-modal training, a finding consistent with the hypothesis above. 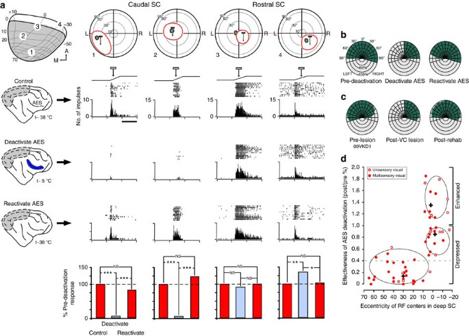Figure 4: AES deactivation differentially modulates deep SC visual activity in rehabilitated animals. (a) Shown are the four recording sites in the ipsilesional rehabilitated SC and the corresponding visual RF (red ovoids) of four (1–4) deep SC neurons. Grey ovoids indicate corresponding superficial RFs. Light bar movement through RF is represented by ramp above response rasters and histograms. Each trial consisted of 10 stimulus presentations; interstimulus interval 30 s. The neurons’ responses to the three experimental conditions (control, deactivate AES, reactivate AES) are shown, with the per cent of response modulation plotted in the bar graphs. Pairedt-test. *P<0.01; **P<0.001; ***P<0.0001; NS, not significant. Note that AES deactivation produced various effects, ranging from profound depression (that is, neurons 1 and 2) to no significant change (that is, neuron 3) to enhancement (that is, neuron 4). Scale bar, 1 s. (b) After completing of electrophysiological experiments, visual orientation capabilities were evaluated before, during and following AES deactivation. Right AES deactivation during the task reinstated contralateral anopia, consistent with the attenuation of ipsilesional SC visual activity observed during the recording experiments (a). Similarly, AES reactivation reinstated visual orientation in the anopic hemifield, mirroring the re-emergence of activity in the deep SC. (c) Loss and re-emergence of visual orientation competencies during AES deactivation/reactivation recapitulated the behavioural sequella observed in this animal during orientation testing, before, and following, cross-modal rehabilitation. (d) Scatter diagram illustrating the effects of AES deactivation on visual responses as a function of RF eccentricity observed in deactivation experiments (n=2). K-means cluster analysis revealed three distinct populations that were differentially distributed in the SC. Ellipsis delimits 95% confidence levels for each population, with the individual population mean denoted by +. The greatest response attenuation during deactivation was seen in neurons representing regions of visual space rendered anopic by cortex lesions. By contrast, neurons representing central visual space (and largely unaffected by visual cortex lesions) were either modestly affected or were enhanced by AES deactivation. Although both unisensory visual (open circles) and visual-multisensory (closed circles) neurons were both affected, most were multisensory. Horizontal dashed line indicates the maximum attenuation of visual responsiveness reported previously in intact animals (29), indicating that AES has a more profound influence on deep SC visual activity in rehabilitated animals. Figure 4: AES deactivation differentially modulates deep SC visual activity in rehabilitated animals. ( a ) Shown are the four recording sites in the ipsilesional rehabilitated SC and the corresponding visual RF (red ovoids) of four (1–4) deep SC neurons. Grey ovoids indicate corresponding superficial RFs. Light bar movement through RF is represented by ramp above response rasters and histograms. Each trial consisted of 10 stimulus presentations; interstimulus interval 30 s. The neurons’ responses to the three experimental conditions (control, deactivate AES, reactivate AES) are shown, with the per cent of response modulation plotted in the bar graphs. Paired t -test. * P <0.01; ** P <0.001; *** P <0.0001; NS, not significant. Note that AES deactivation produced various effects, ranging from profound depression (that is, neurons 1 and 2) to no significant change (that is, neuron 3) to enhancement (that is, neuron 4). Scale bar, 1 s. ( b ) After completing of electrophysiological experiments, visual orientation capabilities were evaluated before, during and following AES deactivation. Right AES deactivation during the task reinstated contralateral anopia, consistent with the attenuation of ipsilesional SC visual activity observed during the recording experiments ( a ). Similarly, AES reactivation reinstated visual orientation in the anopic hemifield, mirroring the re-emergence of activity in the deep SC. ( c ) Loss and re-emergence of visual orientation competencies during AES deactivation/reactivation recapitulated the behavioural sequella observed in this animal during orientation testing, before, and following, cross-modal rehabilitation. ( d ) Scatter diagram illustrating the effects of AES deactivation on visual responses as a function of RF eccentricity observed in deactivation experiments ( n =2). K-means cluster analysis revealed three distinct populations that were differentially distributed in the SC. Ellipsis delimits 95% confidence levels for each population, with the individual population mean denoted by +. The greatest response attenuation during deactivation was seen in neurons representing regions of visual space rendered anopic by cortex lesions. By contrast, neurons representing central visual space (and largely unaffected by visual cortex lesions) were either modestly affected or were enhanced by AES deactivation. Although both unisensory visual (open circles) and visual-multisensory (closed circles) neurons were both affected, most were multisensory. Horizontal dashed line indicates the maximum attenuation of visual responsiveness reported previously in intact animals (29), indicating that AES has a more profound influence on deep SC visual activity in rehabilitated animals. Full size image To determine if AES deactivation would have comparable effects on visual orientation after rehabilitation, one of these physiologically evaluated animals underwent AES deactivation while performing the visual orientation task. As expected, visual cues delivered in the recovered hemifield failed to evoke orientation during AES deactivation, recapitulating the deficit seen before rehabilitation ( Fig. 4b ). By contrast, visual cues presented in the opposite hemifield evoked robust visual orientation ( Fig. 4c ). Taken together, the data indicate that a new functional cortical–midbrain relationship had been established by the cross-modal training, one that was now capable of supporting visuomotor behaviours in the absence of visual cortex. To determine whether the reinstated visuomotor competencies could be used for more than the simple detection and localization of visual cues, rehabilitated animals ( n =2) were challenged with forced-choice discrimination tasks ( Fig. 1d ) that required the discrimination of the features of the visual test cues. The first task involved discriminating vertical from horizontal striations. Both animals learned to perform this task to the same performance levels they exhibited before the cortical lesion at the four lowest spatial frequencies tested (0.28; 0.4; 1.0; 2.0 Hz) although they began to fail at higher frequencies (3.0 and 4.0 Hz, Fig. 5a ). One of these animals was then trained on a second task that involved discriminating among objects. It was able to learn to reliably discriminate an upright from an inverted triangle and a cross from an annulus, although with lower performance than it exhibited pre-operatively ( Fig. 5b,c ). These observations indicate that the rehabilitated circuitry was capable of appreciating complex features of the visual scene. 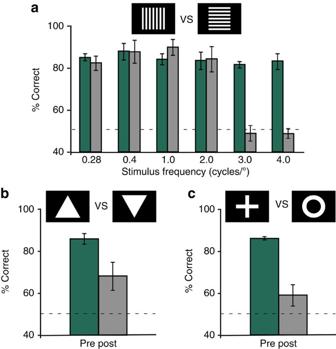Figure 5: Visual discriminative capabilities of rehabilitated animals. This animal was trained in the orientation task as well as three forced-choice visual discrimination tasks (vertical versus horizontal gratings; upright versus inverted triangle; cross versus annulus) before visual cortical extirpation. Pre-lesion capabilities are shown in green; post-cross-modal training performance in grey. (a) Before visual cortex removal, the animal performed the spatial frequency task with a high level of proficiency. It performed well above the chance levels, discriminating vertical versus horizontal gratings at spatial frequencies up to the limit tested (4.0 cycles/°). By contrast, after cross-modal training and the reinstatement of visual orientation behaviours, the animal reacquired the ability to discriminate such stimuli albeit never achieving the previous level of proficiency as discriminations of the highest levels tested (3.0, 4.0 c/d) fell to chance levels. Each bar represents performance on four consecutive testing days of 100 trials per day. Error bars represent s.d. (b,c) Similarly, performance with more complex stimuli (triangle orientation; cross versus annulus) was above chance levels after cross-modal training but also failed to achieve pre-lesion levels. Pre- and post bars inbrepresents performance on 4 and 13 consecutive testing days of 100 trials/day, respectively. Pre- and post bars increpresents performance on 5 and 9 consecutive testing days of 100 trials per day, respectively. Error bars represent s.d. These data indicate that cross-modal training facilitates the reacquisition of previously learned feature discriminations. Figure 5: Visual discriminative capabilities of rehabilitated animals. This animal was trained in the orientation task as well as three forced-choice visual discrimination tasks (vertical versus horizontal gratings; upright versus inverted triangle; cross versus annulus) before visual cortical extirpation. Pre-lesion capabilities are shown in green; post-cross-modal training performance in grey. ( a ) Before visual cortex removal, the animal performed the spatial frequency task with a high level of proficiency. It performed well above the chance levels, discriminating vertical versus horizontal gratings at spatial frequencies up to the limit tested (4.0 cycles/°). By contrast, after cross-modal training and the reinstatement of visual orientation behaviours, the animal reacquired the ability to discriminate such stimuli albeit never achieving the previous level of proficiency as discriminations of the highest levels tested (3.0, 4.0 c/d) fell to chance levels. Each bar represents performance on four consecutive testing days of 100 trials per day. Error bars represent s.d. ( b , c ) Similarly, performance with more complex stimuli (triangle orientation; cross versus annulus) was above chance levels after cross-modal training but also failed to achieve pre-lesion levels. Pre- and post bars in b represents performance on 4 and 13 consecutive testing days of 100 trials/day, respectively. Pre- and post bars in c represents performance on 5 and 9 consecutive testing days of 100 trials per day, respectively. Error bars represent s.d. These data indicate that cross-modal training facilitates the reacquisition of previously learned feature discriminations. Full size image The present experiments revealed that the contralesional haemianopia induced by large unilateral visual cortex lesions, and the accompanying loss of visual responsiveness in the deep (for example, multisensory) layers of the ipsilesional SC, can be reversed by a simple cross-modal training paradigm. The striking rehabilitative effects that were induced by training with spatiotemporally concordant auditory and visual stimuli were linked to changes in the descending tectopetal influences from association (that is, AES) cortex, changes that rendered their target SC neurons once more capable of transforming visual cues into appropriate orientation behaviours. That such cross-modal training can affect visual function is consistent with observations from previous studies. For example, it has been shown that visual–auditory training promotes the learning of both unisensory visual, and unisensory auditory tasks (see, for example, refs 27 , 28 , 29 ) and can do so in individuals with impaired sensory functions (see, for example, refs 30 , 31 ). Furthermore, concurrent auditory–visual stimulation enhances the detection and localization of suboptimal visual stimuli [32] , [33] , [34] , [35] , [36] , [37] and, consistent with the principle of inverse effectiveness [38] , does so most strongly when the visual stimuli involved are least effective [14] . However, it is surprising to note that training with a single contralesional location induced rehabilitation throughout the previously anopic hemifield in a central-to-peripheral fashion. It will be of interest to determine whether training with multiple contralesional loci would enhance the speed of rehabilitation by activating a wider set of collicular inputs or whether it would compromise this process by decreasing the incidence of cross-modally activated neurons in a given location and/or by the introduction of ambiguity [39] . The involvement of AES cortex in this recovery process also is consistent with its normal role of integrating, and thereby enhancing, the sensory responses of multisensory SC neurons [6] . The visual and auditory subdivisions of AES send substantial converging projections onto individual neurons in the ipsilateral SC [40] , [41] that provide the synergistic influences needed to engage in multisensory response enhancement [26] . In the absence of inputs from association cortex, SC multisensory neurons respond to visual–auditory cues by averaging their individual influences, and thereby responding less robustly than they would to the best unisensory input alone, or by responding as if only one of the cues were present [26] . Thus, one likely possibility is that the residual visual inputs, initially too weak to drive the postsynaptic SC neuron, are strengthened by cross-modal training via Hebbian-like mechanisms (via the AES-SC projection), so that once again, such stimuli can engage its visuomotor role. That neurons in the auditory and visual regions of AES are highly sensitive to experience with these two sensory modalities has been repeated demonstrated, revealing that their individual representations can expand or contract dynamically based on the relative level of modality-specific experience [25] , [42] , [43] , [44] . That these physiological changes are, in turn, related to SC function is suggested by the associated changes in the animal’s overt orientation and localization capabilities [24] , [45] , [46] . Presumably, cross-modal training provides the AES with the ability to facilitate deep SC responsiveness not only via its own intrinsic visual activity (which is likely to have been seriously compromised by the loss of its inputs from extrastriate visual cortex [47] ), but also by enhancing the effectiveness of other visual inputs coming directly from the retina [48] or indirectly from the superficial SC [49] , [50] . As the current findings reveal, superficial layer SC neurons remained visually responsive following these extensive visual cortex lesions. Such neurons are likely to be the most substantial remaining source of visual input to AES (via ascending thalamic projections to the lateral posterior/pulvinar complex [51] and to deep layer multisensory neurons [49] , [50] . Modulation of afferents to the SC is believed to be a hallmark of the AES component of this visuomotor circuit in the normal brain [52] , [53] , [54] , and AES appears to retain this role after visual cortex lesions. Indeed, it is critical for the rehabilitative effects noted here. The ascending SC-lateral posterior/pulvinar projections from the SC also may play a significant role in discriminative capabilities observed following cross-modal rehabilitation. Consistent with this possibility are recent findings that superficial SC neurons perform more sophisticated visual analyses than previously thought [55] and that such projections via these thalamic nuclei are likely to be involved in human blindsight [56] , [57] . That AES also projects to other collicular-related structures suggests that the compensatory plasticity that follows cross-modal training may not be limited to alterations of direct AES-SC projections. For example, we have noted previously that the SC’s role in visuomotor behaviours is best appreciated by considering its intimate anatomical and physiological relationships with the basal ganglia [58] , [59] , structures widely regarded as crucial for action selection and reinforcement learning [60] . The involvement of the basal ganglia in ameliorating haemianopia is evident from previous studies whereby manipulations of its projections to the deep SC reverses haemianopia [61] , presumably by altering a pathway critical for the bilateral coordination of midbrain visuomotor activity [62] . Given that the basal ganglia also receives direct projections from AES [51] , [63] , understanding how cross-modal training impacts this broader architecture will likely provide additional insights into its underlying mechanisms. Of particular concern in future studies is how cross-modal training achieves a proper balance among the components of this architecture that is necessary to produce the coordinated visuomotor behaviours observed here. Yet, the fact that it does, suggests that despite the progressive encephalization of visual function that occurred during mammalian evolution [64] , [65] , phylogenetically older circuits retain their ability to support sophisticated visual behaviours. It is highly likely that similar mechanisms also contribute to the visual search improvements in human haemianopic patients following cross-modal training [31] . Adult mongrel cats ( n =23) of both sexes and ranging from 1.5 to 7 years of age were used. Animals were obtained from a USDA-licensed commercial animal breeding facility (Liberty Labs, Waverly, NY). All procedures were performed in compliance with the 8th Edition of the ‘Guide for the Care and Use of Laboratory Animals’ (National Research Council of the National Academies, 2011) and approved by the Institutional Animal Care and Use Committee (IACUC) at Wake Forest School of Medicine. All efforts were made to minimize the number of animals used and to alleviate any discomfort. Twenty animals exhibited enduring deficits, as defined by the absence of recovery after a minimum of a 2.5-month period in a normal visual environment, which were induced by complete removal of all contiguous regions of visual cortex. These animals formed the sample used in the experiments described below. In an additional three animals, the posterior aspect of the AES was removed. Pre- and post-operative visual orientation testing Visual orientation capabilities were evaluated in a semicircular orientation arena [17] . The arena was subdivided into 15° sectors, extending from 105° left to 105° right. Visual test cues (white ping-pong ball on the end of a wire wand) were delivered manually, emerging suddenly from behind a black curtain hung parallel to the black arena walls ( Fig. 1a ). The curtain minimized extraneous visual cues associated with stimulus delivery and eliminated anticipatory movements. Food-restricted animals were gently restrained by a handler so that its head and eyes were directed towards the 0° fixation mark, 58 cm away. The handler was blind to the location of test cues. Animals were trained to fixate directly ahead on a food reward held by forceps that protruded through a hole in the apparatus’ front wall. A trial began when the experimenter, who monitored the animals’ head/eye position, determined that they were fixating and gave the verbal command ‘Go’. At that time, animals were released and moved towards the 0° fixation point for a food reward. On test trials, the visual stimulus emerged from behind the curtain coincident with the Go command. If the animal oriented towards the cue, a food reward was delivered at cue location. If the animals did not orient to the test cue, or if no cue was delivered (that is, ‘catch’ trials), they moved ahead to receive a food reward. These quasi-randomly presented catch trials effectively minimized scanning and ‘false’ responses. Cue delivery locations were assigned quasi-randomly at 15° eccentricities along the horizontal meridian. Typically, each eccentricity was tested four times in each session. After a variable period of training, intact animals responded to stimulus delivery on nearly every trial, albeit with somewhat lowered accuracy at the most peripheral locations. Criterion performance was an average of 95% correct responses throughout the visual field. Typically, a minimum of 100 stimulus presentations was delivered at each eccentricity. Before each testing session, animals were food restricted for 24 h with free access to water. Testing was conducted Monday–Friday at approximately the same time of day for each animal. If the daily food ration was not consumed during testing, the remainder of the ration was provided in the testing environment. Animals were fed their allotted daily ration over weekends. Weekly charting revealed stable weight profiles. Post-operative cross-modal training Cross-modal training was conducted in the same arena used for visual orientation testing (see above). Post-ablation animals displaying a stable and persistent deficit (operationally defined as a minimum of 2.5 months of contralesional haemianopia) were initially rewarded for orienting to the sound of the ping-pong ball rubbed down and against the vertical wall of the testing arena ( Fig. 1b ). Thus, the rehabilitative stimulus consisted of an (effective) auditory cue (≈70 dB against a ≈50 dB background) combined with an ineffective, albeit spatially and temporally coincident, visual cue. Once animals reliably oriented to this cross-modal stimulus, rehabilitative training began. The task required animals to fixate ahead and then orient to and approach the test cue. There were three conditions—the cross-modal cue appeared at 45° in the anopic hemifield; the visual cue appeared alone at the equivalent position in the functional hemifield; and the ‘catch’ trial. The daily ratio of cue in the anopic hemifield (cross-modal), the functional hemifield (visual only) and the catch trial condition was ∼ 45:15:10. Rehabilitative sessions were conducted 5 days per week (Monday–Friday) or, in select animals, 7 days per week for a period of 4 weeks. The progressive recovery was monitored during rehabilitation with visual-only probing trials in the anopic hemifield immediately following each session. In some animals, the probe trials also were conducted a second and third time, ∼ 60 min later and again immediately before the subsequent training session on the following day. As in the initial visual orientation training procedure, animals were food-restricted for 24 h before a rehabilitative session with free access to water. On completion of rehabilitative training, animals were evaluated in the standard visual orientation task for a minimum of 2 months to verify the persistence of the recovered function. Auditory rehabilitation control To determine whether an auditory cue alone was sufficient for rehabilitation, select animals ( n =2) were trained with only the auditory cue in the anopic hemifield. Testing was conducted in a matte black semicircular perimetry arena, 116 cm in diameter and bounded by 60 cm high walls ( Fig. 1c ). Speakers and red light emitting diodes (LEDs) were mounted in the arena’s wall at 15° intervals. Speaker grill cloth covered the wall, minimizing visual heterogeneities. Speakers (Kobitone part #25CE500- RO; Mouser Electronics, Mansfield, TX) were 3.8 cm in diameter with a frequency response of 20 Hz–20 KHz. They were located 58 cm from the animal’s start position and at approximately the pinnae height. Speakers delivered computer-generated white noise bursts 100 ms in duration and 70±2 dB in intensity, so that their parameters approximated those of the cross-modal rehabilitative cue. Acoustic calibration was conducted with sound level metre (Model 1800, Quest Technologies, Oconomowoc, WI) with a microphone placed equidistant between the left and right speakers. Mean ambient noise was ≈50 dB, and auditory test cues were presented 20 dB above this background. LED’s delivered computer-controlled light pulses (250 ms duration; 0.48 m.c.d. intensity. All testings were conducted in a dimly lit room, and the task structure and probe testing were identical to that in cross-modal training. There were three conditions—cross-modal cue appeared at 45° in the anopic hemifield; visual cue appeared alone at the equivalent position in the functional hemifield; and ‘catch’ trials. The daily ratio of cues in the anopic hemifield (cross-modal); the functional hemifield (visual only); and the catch trial condition was ∼ 45:15:10. Feature discrimination To determine whether rehabilitated animals also possessed any other fundamental visual capabilities, animals ( n =2) were trained before visual cortex ablation in a two forced-choice task to discriminate horizontal versus vertical gratings of varying spatial frequencies. Testing was conducted in a matte black arena, 120 × 120 × 60 cm with a pair of 19 inch computer monitors positioned 57 cm from the animal’s initial position and 20° eccentric to its central fixation ( Fig. 1d ). Discriminanda were generated by custom designed software (Visual Basic, Microsoft, Redmond, WA). Food-restricted animals were manually restrained and required to fixate on a LED positioned directly ahead for 2 s or more, and on stable fixation, paired discriminanda were presented on the monitors. One stimulus was selected as the positive discriminanada, and animals orienting towards and approaching the appropriate screen received a food reward on a tray beneath the screen. The vertical-horizontal gating consisted of a 10.5 × 10.5 cm array of alternating black and white bars of various widths (2, 1.5, 0.75, 0.5, 0.25, 0.125 cm), yielding spatial frequencies at fixation viewing angles of 0.28, 0.4, 1.0, 2.0, 3.0, 4.0 cycles/°. One animal was further trained to discriminate (i) an inverted versus an upright triangle (white equilateral triangles, base width 10.5 cm) and (ii) a white cross (base width 10.5 cm) versus a white annulus (diameter 10.5 cm, line width 2 cm with similar total luminance. Positive and negative discriminanda were shifted from left to right viewing screens according to a random number generator. Selection of ablation laterality Because visual orientation performance to more peripheral visual cues (that is, 90°, 105°) was typically better in one hemifield than the other, the hemisphere representing the higher performance hemifield was always selected for extirpation. To facilitate comparisons, all data presented were normalized to represent right hemisphere ablation/left visual fields. In each case, the performance in the non-optimal hemifield improved for peripheral stimuli following visual cortex ablation and became as good as, and typically better than, that seen before ablation. Surgical procedures for visual cortex ablation All surgery was conducted aseptically. Animals were administered dexamethasone (1 mg kg −1 , intramuscular (i.m.)) perioperatively to minimize cerebral edema. Animals were anaesthetized with pentobarbital sodium (22–30 mg kg −1 , intraperitoneal (i.p.)) to replicate experimental conditions used previously [2] , [3] . This is critical because anaesthetic agents can influence the appearance of visuomotor deficits following visual cortex lesions [17] . On cessation of corneal blink reflexes, animals were placed in a stereotaxic head-holder, and an endotracheal tube was inserted for artificial ventilation. Animals were placed on a heating pad, and the saphenous vein was catheterized. Core body temperature, expiratory CO 2 , blood pressure and heart rate were monitored (SurgiVet Advisor, Smith Medical, Dublin, OH, USA) and maintained within normal physiological bounds. The surgical site was shaved and scrubbed with betadine. A midline scalp incision was made, and a craniotomy exposed the cortical areas to be removed. After reflecting the dura, the grey matter was extirpated by subpial aspiration. Approximately, the posterior three-fourths of the lateral and suprasylvian gyrus and a portion of the posterior ectosylvian gyrus were removed. The grey matter of the medial aspect of the hemisphere posterior to the cruciate gyrus was removed above the splenial sulcus. Thus, the following cortical areas were removed—17, 18, 19, 20a, 20b, 21a, 21b, DLS, VLS, PS, PMLS, PLLS, AMLS, ALLS, 5, 7 and SVA [66] . In all cases, the initial lesion spared the AES, thereby sparing its visual and visual-multisensory representations. Following ablation, the aspiration defect was packed with gelfoam, the cranial bone plate replaced and the scalp incision closed with sutures. Prophylactic doses of analgesics (ketoprofen 2 mg kg −1 , i.m.) and antibiotics (cefazolin, 20 mg kg −1 , i.m.) were administered post-operatively. Physiological saline (50–200 ml, subcutaneous (s.c.) or intravenous (i.v.)) was administered to compensate for insensate fluid loss. Animals recovered in a lighted environment to maximized the likelihood of creating a permanent deficit [67] . Animals were monitored post-operatively until the return of sternal recumbence and active locomotion, after which they were returned to their home cage. Analgesia was provided within the first 24 h and continued, if required, as long as necessary based on signs of distress. Immediately following recovery from anaesthesia, all animals displayed marked tonic ipsiversive head deviation and ipsiversive circling behaviour, which resolved gradually within 1–2 days. Neurological evaluation during this time revealed a lack of blink-to-threat reflex for contralesional stimuli, with no indication of orientation to visual cues presented at any position within the contralesional hemifield. Responses to contralesional tactile stimuli were usually preserved but attenuated. Contralesional auditory orientation deficits were present but resolved within the first post-operative week. Blink-to-threat deficits and visual haemianopia remained. Surgical techniques for electrophysiological recordings All surgeries were conducted aseptically. Animals were administered dexamethasone (1 mg kg −1 , i.m.) perioperatively to minimize cerebral oedema. Animals were pre-anaesthetized with ketamine hydrochloride (20–30 mg kg −1 , i.m.) and acepromazine maleate (0.05–0.1 mg kg −1 , i.m.) and placed in a stereotaxic head-holder. Following intubation, animals were artificially ventilated, and anaesthesia was maintained with inhalation of isofurane (0.5–4.0%). Expiratory CO 2 was monitored, and respiration rate and/or volume adjusted to maintain the expired CO 2 within the range of 3.5–4.5%. Heart rate and blood pressure were monitored to ensure surgical plane of anaesthesia. Core body temperature was monitored rectally and maintained at normal levels with a heating pad. The eyes were covered with a topical ophthalmic ointment to prevent corneal drying and to minimize the chance of conjunctival infection. The scalp was incised, and bone removed from the calvarium with a high-speed bur to access to SC and/or AES. A stainless steel recording well/head-holder was fitted to facilitate recordings [68] . In select animals, a stainless steel cryogenic deactivation coil [22] also was implanted into the AES sulcus. A micro-thermistor (IT-23—Physitemp Instruments, Inc, Clifton, NJ) for monitoring cortical temperature during thermal deactivation was fitted to the tubing during fabrication. The tubing was run to the top of the skull where the ends terminated within a stainless steel chamber that was affixed to the skull with bone screws and cement. Four tungsten recording electrodes also were implanted near the cooling coil to directly monitor AES neural activity during thermal deactivation. All hardware was anchored to the skull with stainless steel screws and dental acrylic. Prophylactic doses of analgesics (ketoprofen 2 mg kg −1 i.m. ), antibiotics (cefazolin, 20 mg kg −1 , i.m.) and dexamethasone were administered post-operatively. Physiological saline (50–200 ml, s.c. or i.v.) was administered to compensate for insensate fluid loss. Animals were monitored post-operatively until the return of sternal recumbency and active locomotion, after which they were returned to their home cage. Analgesia was provided within the first 24 h and continued as required. The first recording sessions were not conducted until a minimum of 10–14 days post implantation. Cortical cryogenic deactivation techniques Cortical deactivation was accomplished via indwelling coils placed between the sulcal walls of AES as described previously [22] . The cooling coils were fabricated by fashioning loops of 20–21 gauge stainless steel hypodermic tubing that are shaped appropriately for the sulcus. Iced water (≈0 °C) was circulated through the coils to decrease cortical temperature to ≈10 °C to deactivate the cortex, and the cortex was allowed to rewarm passively to 36–38 °C. Coil stems were fixed to the skull with surgical screws and orthopaedic cement. Miniature thermocouples (Omega Engineering, Stamford, CT) were implanted in cortex adjacent to the probes to measure temperature. Physiological monitoring confirmed the attenuation and return of cortical activity. Previous studies showed that this technique induces no apparent damage to underlying neurons and produces a limited area of cortical deactivation that is restricted to AES [22] . Procedures for electrophysiological recordings Anaesthesia was induced with an initial bolus of ketamine HCl (20–30 mg kg −1 , i.m.) and acepromazine (0.2 mg kg −1 , i.m.). The animal’s head was secured during the recording session by attaching the implanted head-holder to the stereotaxic frame, thereby providing painless support without the presence of pressure points or obstruction of the eyes [68] . The saphenous vein was catheterized for i.v. fluid administration. Following endotracheal intubation, neuromuscular blockage was induced with either pancuronium bromide (0.04–0.1 mg kg −1 , i.v.) or rocuronium bromide (0.5–0.7 mg kg −1 , i.v.) to prevent ocular drift, and the animal was artificially respired. End tidal CO 2 was monitored and maintained at ∼ 4.0% by manipulating inspiration rate and/or volume. Core body temperature was maintained using a heating pad. A constant infusion of ketamine HCI (2–5 mg kg −1 per h) sufficient to maintain anaesthesia in non-paralysed preparations was delivered intravenously, along with pancuronium bromide (0.05 mg kg −1 per h) or rocuronium bromide (0.1 mg kg −1 per h) and 5% dextrose in 0.9% saline (3–6 ml h −1 ). Pupils were dilated with 1% atropine sulfate, and the nictitating membranes and eyelids were retracted with 2.5% phenylephrine hydrochloride. The refractive state of each eye was measured by direct ophthalmoscopy, and contact lenses of the appropriate powers were fitted to focus the eyes on a translucent Plexiglas hemisphere positioned in front of the animal. The positions of the optic disc and area centralis were plotted onto the dome by means of reverse ophthalmoscopy. Vital signs (for example, heart rate, blood pressure, end tidal CO 2 , core body temperature, pCO 2 ) were monitored (SurgiVet Advisor, Smith Medical, Dublin, OH). Anaesthetic levels under neuromuscular blockade were assessed in accordance with IACUC approved protocols. Blood pressure and heart rate were continuously monitored, and ketamine hydrochloride infusion rates were manipulated as required to insure that these physiological parameters did not deviate significantly from values normally seen under ketamine anaesthesia alone. After the recording session, paralytics were discontinued, and, on restoration of normal respiration, anaesthesia was terminated. Following stable locomotion, animals were returned to their home cage. Extracellular recordings were made with epoxylite insulated tungsten microelectrodes (2–4 MΩ). Neuronal responses were band-pass amplified, displayed on an oscilloscope, fed into a window discriminator and subsequently routed to computer disc using a 1401+ hardware acquisition system (CED Systems, Cambridge, England) running CED Spike2 software. Visual RF mapping and initial qualitative evaluation of neuronal response properties were made using spots or bars of light projected from a hand-held ophthalmoscope. Neurons also were evaluated for responses to non-visual (that is, auditory and/or somatosensory) stimuli using manually delivered auditory (claps, clicks, finger snaps) and tactile (taps, brushes) stimuli. For quantitative assessment, light stimuli of various shapes and sizes were projected onto the hemisphere via an electronically controlled, galvanometer-driven mirror system and auditory stimuli (broadband noise bursts: 100 ms duration, 70 dB) were delivered from a moveable speaker. The stimuli were presented repeatedly ( n =10–16 times per test, at 6–10 s intervals) within the appropriate RF. Histological evaluation of cortical lesions Following data collection, animals were sedated with ketamine hydrochloride (20 mg kg −1 , i.m.) and, following the loss of pinna reflexes, injected with lethal doses of pentobarbital (100 mg kg −1 , i.p.). They then were exsanguinated by transcardial perfusion with 0.9% saline followed by 4% paraformaldehyde fixative. Brains were removed, photographed, cut on a cryostat and processed using routine histological procedures. The extent of each cortical lesion was determined by charting the damage in serial coronal sections with post-fixation photographs of the brain. The reconstructed lesion then was correlated to standard physiological and anatomical maps to assess its extent [66] . Microscopic examination of neutral red-stained sections through the dorsal lateral geniculate nucleus documented the extent of retrograde degeneration. How to cite this article : Jiang, H. et al . Multisensory training reverses midbrain lesion-induced changes and ameliorates haemianopia. Nat. Commun . 6:7263 doi: 10.1038/ncomms8263 (2015).